Topological states in a ladder-like optical lattice containing ultracold atoms in higher orbital bands Topological insulators are classified according to their symmetries. Discovery of them in electronic solids is thus restricted by orbital and crystalline symmetries available in nature. Synthetic quantum matter, such as the recent double-well optical lattices loaded with s and p orbital ultracold atoms, can exploit symmetries and interaction beyond natural conditions. Here we unveil a topological phase of interacting fermionic atoms on a two-leg ladder derived from the above experimental optical lattice by dimension reduction. The topological band structure originates from the staggered phases of sp orbital tunnelling, requiring neither spin–orbit coupling nor other known mechanisms like p -wave pairing, artificial gauge field or rotation. Upon crossing over to two-dimensional coupled ladders, the edge modes from individual ladder form a parity-protected flat band at zero energy. Experimental signatures are found in density correlations and phase transitions to trivial band and Mott insulators. Novel lattice geometries have been known to give rise to interesting many-body phenomena including topological states of quantum matter. In the context of ultracold quantum gases, optical lattices engineered with interfering laser beams can realize specific configurations of potentials of single or multiple periods not found in nature. For instance, double-well superlattices [1] , [2] have matured into a powerful tool for manipulating orbital degrees of freedom [3] , [4] , [5] , [6] , [7] , [8] , [9] , [10] . Controls of atoms in the s and p orbitals of the checkerboard [6] and hexagonal [8] optical lattices have also been demonstrated, and correlation between these orbitals tends to give exotic quantum states [6] , [8] , [11] , [12] , [13] . The spatial symmetry of the orbital wavefunction dictates the complex hopping amplitudes between nearby sites. Under certain circumstances, as for the uneven double wells, the orbital hopping pattern is sufficient for producing topologically nontrivial band structures [14] . Motivated by these developments, here we consider a lattice of uneven double wells where fermionic atoms are loaded up to the s and p orbital levels of the shallow and deep wells, respectively. This new configuration of orbitals beyond solid state materials realizes a topological band insulator phase of interacting fermions with edge states. Topological phase transitions to trivial band and Mott insulators are predicted as a feature of the topological state. Remarkably, the edge states persist upon dimensional crossover, which makes it promising to realize in optical lattice experiments. This route of achieving topological band insulators and superfluids is distinct from previous proposals that require rotation of the gas [15] , [16] , artificial gauge fields [17] , spin–orbital coupling [18] , [19] , [20] , [21] or p -wave triplet pairing [22] . One-dimensional orbital ladder We will first focus on a one-dimensional (1D) ladder system illustrated in Fig. 1b . 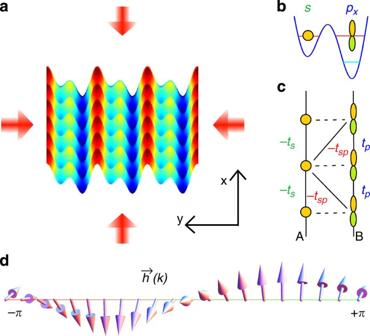Figure 1: Thesporbital ladder reduced from a 2D double-well optical lattice. (a) An optical lattice of uneven sub-wells (light and dark blue), with parametersVx/V1=0.3,V2/V1=1 andφ=0.6π, develops high barriers (red ridges) in theydirection, slicing the lattice into dynamically decoupled uneven two-leg ladders. (b,c) Schematic side and top views, respectively, of the ladder illustrate tunneling (t′s) of fermions prepared in the degeneratesandpxlevels. (d) Topological winding of Hamiltonian across the Brillouin zone. This corresponds to the quasi-1D limit of a standard double-well optical lattice, with the optical potential given by Figure 1: The sp orbital ladder reduced from a 2D double-well optical lattice. ( a ) An optical lattice of uneven sub-wells (light and dark blue), with parameters V x / V 1 =0.3, V 2 / V 1 =1 and φ =0.6 π , develops high barriers (red ridges) in the y direction, slicing the lattice into dynamically decoupled uneven two-leg ladders. ( b , c ) Schematic side and top views, respectively, of the ladder illustrate tunneling ( t ′s) of fermions prepared in the degenerate s and p x levels. ( d ) Topological winding of Hamiltonian across the Brillouin zone. Full size image This optical lattice has a double-well structure in the y direction. For V 1,2 >> V x , there is a large tunnelling barrier between double wells in the y direction, so in low-energy physics the two-dimensional (2D) system decouples into an array of dynamically isolated two-leg ladders of A and B sub-wells ( Fig. 1 ), with each ladder extending in the x direction. The relative well depth of the two legs is controlled by the phase φ and further by the ratio V 2 / V 1 . We will focus on a situation, similar to the setup in the experiment [6] , where the s orbital of leg A has roughly the same energy as the p x orbital of leg B (other p orbitals have much higher energy). For example, one can choose V 1 =40 E R , V 2 =20 E R , V x =4.0 E R and φ =0.9 π in experiments, where E R is the recoil energy , with m the mass of atom and k the wave number of the laser. Such a setup will give the A (B) wells a depth 2.7 E R (8.1 E R ). The tunnelling rates of the various orbitals illustrated in Fig. 1c are given as t s =0.053 E R , t p =0.40 E R and t sp =0.064 E R in the tight binding approximation. The lattice constant a = π / k will be set as the length unit in this paper. We now consider a single species of fermions occupying these orbitals, with the low-lying s orbital of leg B completely filled. Alternatively fermions can be directly loaded into the p x orbital of leg B, leaving the low-lying s empty, by techniques developed in recent experiments [4] , [6] , [10] . With these techniques, long-lived meta-stable states of atoms in high orbitals with life time on the order of several hundred milliseconds are demonstrated achievable [6] . The Hamiltonian of the sp orbital ladder is then given by where , with and being fermion creation operators for the s and p x orbitals on the A and B leg, respectively. The relative sign of the hopping amplitudes is fixed by parity symmetry of the s and p x orbital wavefunctions. As depicted in Fig. 1c , the hopping pattern has a central role in producing a topological phase. With a proper global gauge choice, t s , t p and t sp are all positive. The rung index j runs from 0 to L −1 with L the system size. We consider half filling (one particle per unit cell), for which the chemical potential μ =0, and the Hamiltonian is particle-hole symmetric under transformation . Topologically nontrivial band structure of this sp orbital ladder, which shall be shown analytically next, may be heuristically speculated from the following comparison: the staggered quantum tunnelling resembles spin–orbit interaction [18] , [19] , [20] , [21] , [23] , when the s and p orbital states are mapped to pseudo-spin-(1/2) states. Such a staggered tunnelling can also naturally arise in the checkerboard optical lattice already engineered in the experiment [6] by increasing the laser strength in one direction to reach the quasi-1D limit. The physics of the sp orbital ladder is also connected to the more familiar frustrated ladder with magnetic flux [24] , but the sp orbital ladder appears much easier to realize experimentally. Topological band structure and zero energy edge states In the momentum space the Hamiltonian takes a simple and suggestive form, where h 0 ( k )=( t p − t s )cos( k ), h x =0, h y ( k )=2 t sp sin( k ) and h z ( k )=−( t p + t s )cos( k ). Here, is the unit matrix, σ x , σ y and σ z are Pauli matrices in the 2D orbital space. The energy spectrum consists of two branches, with a band gap E g =min(2 t p +2 t s , 4 t sp ), which closes at either t sp =0 or t s + t p =0. An interesting limit that highlights the nontrivial band structure of our model is that when t p = t s = t sp , the two bands are both completely flat. To visualize the topological properties of the band structure, one notices that as k is varied from − π through 0 to + π , crossing the entire Brillouin zone, the direction of the vector winds an angle of 2 π ( Fig. 1d ). The corresponding Berry phase is half of the angle, γ = π (see Supplementary Note 1 ). The orbital ladder Hamiltonian H 0 belongs to the symmetry group in the notation of [25] , as it has both particle-hole and time-reversal symmetry, in addition to the usual charge U(1) symmetry. Therefore, at half filling, it is a topological insulator characterized by an integer topological invariant, in this case the winding number 1, according to the general classification scheme of topological insulators and superconductors [25] , [26] . The nontrivial topology of the ladder system also manifests in existence of edge states. It is easiest to show the edge states in the flat band limit, t s = t p = t sp ≡ t , by introducing auxiliary operators, . Then the Hamiltonian only contains coupling between φ + and φ − of nearest neighbours, but not among the φ + (or φ − ) modes themselves, Immediately, one sees that the operators φ + (0) and φ − ( L −1) at the left and right ends are each dynamically isolated from the bulk, and do not couple to the rest of the system ( Fig. 2a ). These loners describe the two edge states at zero energy. They are the bonding and anti-bonding modes of s and p orbitals, that is, shared by the two rungs of the ladder. For general parameters away from the flat band limit, the wavefunctions of the edge states are found not to confine strictly at j =0 or L −1, but instead decay exponentially into the bulk with a characteristic length scale . For the lattice strength given above, the decay width is estimated to be two to three times of the lattice constant. Only for , which is potentially reachable in experiments, ξ →0, the edge states are completely confined at the edges. For t sp =0, the bulk gap closes and ξ →∞. The analytical expression for the edge state wavefunctions in the general case are discussed in Supplementary Note 2 . The existence of zero energy edge states is also confirmed by numerical calculation as shown in Fig. 2b . 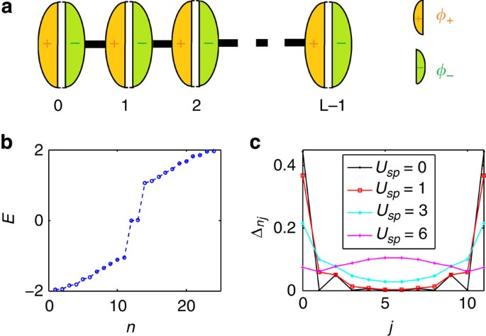Figure 2: Bulk and edge eigenstates of the orbital ladder. (a) A pictorial representation of the simplified Hamiltonian in the flat band limitts=tp=tspshowing the emergence of isolated edge modes. The definition of theφoperator is given in the main text. (b) The eigen energy of a ladder with finite lengthL=12 showing two degenerate zero energy states inside the gap. (c) The probability distribution of the in-gap states (equation (10)) for varying strengths of inter-orbital interactionUsp. The in-gap states are shown localized on the edges and survive against finite interaction. Inbandc, we choosets=tp=2tsp(taken as the energy unit). Figure 2: Bulk and edge eigenstates of the orbital ladder. ( a ) A pictorial representation of the simplified Hamiltonian in the flat band limit t s = t p = t sp showing the emergence of isolated edge modes. The definition of the φ operator is given in the main text. ( b ) The eigen energy of a ladder with finite length L =12 showing two degenerate zero energy states inside the gap. ( c ) The probability distribution of the in-gap states (equation (10)) for varying strengths of inter-orbital interaction U sp . The in-gap states are shown localized on the edges and survive against finite interaction. In b and c , we choose t s = t p =2 t sp (taken as the energy unit). Full size image Fractional charge and topological anti-correlations For a finite ladder of length L with open boundary condition and populated by L fermions (half filling), L −1 fermions will occupy the valence band (bulk states) and one fermion will occupy the edge states ( Fig. 2 ). As the two edge states are degenerate, the ground state has a double degeneracy. The edge state is a fractionalized object carrying half charge (cold atoms are charge neutral, here charge refers to the number of atoms). This becomes apparent if we break the particle-hole symmetry by going infinitesimally away from half filling, for example, tuning chemical potential μ =0 + . Then, the valence band and the two edge states will be occupied. With a charge density distribution on top of the half filled background defined as , one finds , where d satisfies ξ << d << L (for example, take d =5 ξ ). A characteristic feature of the topological insulator (with the number of atoms fixed) is the topological anti-correlation of the charge at the boundaries, In the sharp confinement limit, ξ →0, the edge states are well localized at the two ends of the ladder. The topological anti-correlation simplifies as 〈 ρ (0) ρ ( L −1)〉=−(1/4), and the half charge is also well localized, that is, . As the edge states are well isolated from the bulk states by an energy gap, they are stable against local Gaussian fluctuations. The coupling between the two edge states vanishes in the thermodynamic limit ( L →∞), because the hybridization induced gap scales as exp(− αL ) as L →∞ [27] . Time-reversal symmetry breaking and topological phase transition An interesting topological phase transition to a trivial insulator can be tuned to occur when rotating the atoms on individual sites, for example, by applying the technique demonstrated in [28] . Such an individual site rotation amounts to addition of an imaginary transverse (along y ) tunnelling between s and p x orbitals in our Hamiltonian, This term preserves particle-hole symmetry but breaks both parity and time-reversal symmetries. The total Hamiltonian in the momentum space now reads . This Hamiltonian belongs to the symmetry group G + ( U , C ) and allows a Z 2 classification of its topological properties [25] . Even though time-reversal symmetry is absent, particle-hole symmetry still ensures that Berry phase γ is quantized, with γ mod 2 π =0 or π defining the trivial and topological insulator, respectively [29] . For our model , the topological insulating phase with γ = π is realized as long as . In another word, the Berry phase quantization is robust against the time-reversal symmetry breaking term Δ y , and this topological phase is protected by particle-hole symmetry. For Δ y greater than , Berry phase vanishes and the system becomes a trivial band insulator. At the critical point the band gap closes. Apart from the Berry phase, the topological distinction between and can also be seen from a gapped interpolation [29] as discussed in Supplementary Note 3 . Besides probing the half charges on the boundaries, another signature for the critical point of the topological phase transition is the local density fluctuation, . δρ is 1/ when Δ y =0, independent of other parameters t s , t p and t sp , and decreases monotonically with increasing Δ y (see Supplementary Note 4 ). The peaks of dδρ 2 / d Δ y reveal the critical points ( Fig. 3b ) and provide a reliable tool of detecting the topological phase transition in experiments. 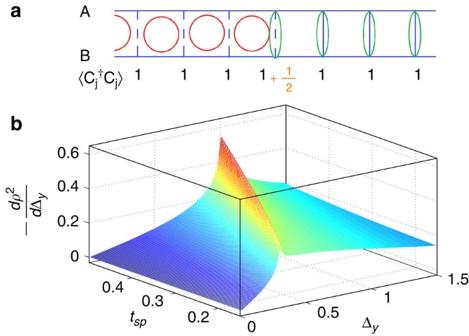Figure 3: Phase transition between topological and trivial band insulators. (a) A domain wall between a topological insulator (ts=tp=tsp, Δy=0, left) and a trivial insulator (ts=tp=tsp=0, right). The circle represents the delocalized fermion shared by two neighbouring rungs as depicted inFig. 2a, whereas the ellipse represents localized fermion without hopping. The additional charge 1/2 in the middle is the fractional charge carried on the domain wall. (b) The derivative of density fluctuation, −(dδρ2/dΔy). It develops sharp peaks, measurable in experiments, along the line of topological critical points. Figure 3: Phase transition between topological and trivial band insulators. ( a ) A domain wall between a topological insulator ( t s = t p = t sp , Δ y =0, left) and a trivial insulator ( t s = t p = t sp =0, right). The circle represents the delocalized fermion shared by two neighbouring rungs as depicted in Fig. 2a , whereas the ellipse represents localized fermion without hopping. The additional charge 1/2 in the middle is the fractional charge carried on the domain wall. ( b ) The derivative of density fluctuation, −( dδρ 2 / d Δ y ). It develops sharp peaks, measurable in experiments, along the line of topological critical points. Full size image It is feasible to prepare the ladder with phase separation: for example, a topological insulator on the left half but a trivial insulator on the right half. This can be achieved by rotating the lattice sites on half of the ladder only. The system is now described by: with a field configuration η ( j ), which satisfies the boundary conditions η ( j =−∞)=0 and η ( j =+∞)= π , and . The charge distribution induced by the domain wall (the phase boundary) is calculated both numerically and from effective field theory shown in Supplementary Note 5 . Both approaches cross-verify that the domain wall carries half charge ( Fig. 3a ). The half charge can be detected [30] by the single-site imaging technique in experiments [31] , [32] . Stability against interactions and transition to a Mott insulator We further examine the stability of the topological phase and its quantum phase transitions in the presence of interaction using exact diagonalization. For single-species fermions on the sp orbital ladder, the leading interaction term is the on-site repulsion between different orbitals, We compute the fidelity metric g as function of the interaction strength U sp (see the Methods section). A peak in the fidelity metric indicates a quantum phase transition [33] . Our numerical results ( Fig. 4 ) show that the topological phase is stable for , with robust in-gap (zero energy) states [33] localized on the edges ( Fig. 2c ). For stronger interaction the ladder undergoes a quantum phase transition to a Mott insulator phase. With t s = t p the Mott state exhibits ferro-orbital order with order parameter defined as (see discussions in Supplementary Note 6 ). Such ferro-orbital order gets weaker as t s gets smaller. A rich phase diagram of orbital ordering is expected and will be investigated in the future. 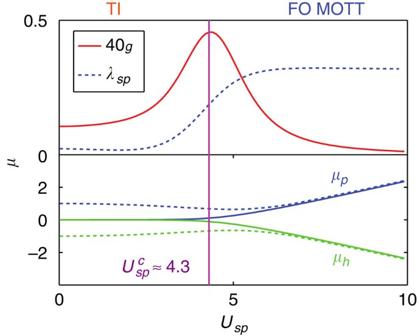Figure 4: Phase transition between topological and ferro-orbital (FO) Mott insulators. Top panel shows the fidelity metricgand the ferro-orbital order parameterλsp, across the transition from the topological insulator (TI) to the Mott insulator. Bottom panel shows the particle/hole chemical potential (μp/μh). The finite charge gapμp−μhin the bulk calculated with periodic boundary condition (dashed lines) comparing with the vanishing gap with open boundary condition (solid lines) indicates in-gap states on the edge. The lengthLis 12, andts=tp=2tsp(taken as the energy unit) in this plot. Figure 4: Phase transition between topological and ferro-orbital (FO) Mott insulators. Top panel shows the fidelity metric g and the ferro-orbital order parameter λ sp , across the transition from the topological insulator (TI) to the Mott insulator. Bottom panel shows the particle/hole chemical potential ( μ p / μ h ). The finite charge gap μ p − μ h in the bulk calculated with periodic boundary condition (dashed lines) comparing with the vanishing gap with open boundary condition (solid lines) indicates in-gap states on the edge. The length L is 12, and t s = t p =2 t sp (taken as the energy unit) in this plot. Full size image Coupled ladders and flat band in two dimensions Remarkably, the zero-energy edge states of the sp orbital ladder survive even when the system is extended to two dimensions with finite inter-ladder coupling (for example, by reducing V 1,2 relative to V x in the setup of Fig. 1a ). The zero modes of individual ladder morph into a flat band with double degeneracy ( Fig. 5 ). The lack of dispersion in the y direction is related to the inter-ladder hopping pattern, which does not directly couple the edge states but only s and p orbitals on different rungs ( Supplementary Fig. 1 ). The unexpected flat band in 2D is an exact consequence of the p orbital parity and hence is protected by symmetry. The flat dispersion can be rigorously proved using an unitary transformation, and arguments based on the quantization of Berry phase in Supplementary Note 7 . The flat band makes the edge states in this 2D optical lattice distinct from that of quantum Hall effect previously proposed with lattice rotation [16] , [34] , artificial gauge field [35] or optical flux [36] . Such a flat band is reminiscent of that at the zigzag edge of graphene, but with the difference that the present flat band is protected by the parity of the orbital wavefunctions. The diverging density of states associated with the flat band provides a fertile ground for interaction-driven many body instabilities. Future work will tell whether strongly correlated topological states exist in such 2D interacting systems. 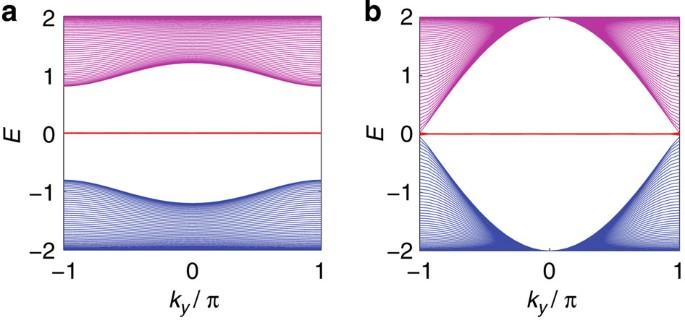Figure 5: Energy spectra of coupled ladders. In this plot we choosets=tp=2tsp(taken as the energy unit here), and lengthL=200. An open (periodic) boundary condition is applied in thex(y) direction.aandbshow the spectra with the small and large inter-ladder coupling,t′sp=tsp/5 andt′sp=tsp, respectively. A flat band (red line) at zero energy with double degeneracy generically appear for 0<t′sp<tsp. Figure 5: Energy spectra of coupled ladders. In this plot we choose t s = t p =2 t sp (taken as the energy unit here), and length L =200. An open (periodic) boundary condition is applied in the x ( y ) direction. a and b show the spectra with the small and large inter-ladder coupling, t ′ sp = t sp /5 and t ′ sp = t sp , respectively. A flat band (red line) at zero energy with double degeneracy generically appear for 0< t ′ sp < t sp . Full size image The mathematical description of the sp orbital ladder H 0 is similar to the celebrated Su-Schrieffer-Heeger (SSH) model [37] . Although the two systems belong to the same symmetry class of 1D topological insulators [25] , the orbital ladder contains new physics beyond the SSH model. First, the edge states of the sp orbital ladder have quite different spatial structures. For example, the sharp confinement of the edge states only requires , rather than the energy spectrum being dispersionless. In contrast, sharp confinement coincides with the flat band limit in the SSH model, when one of its hoppings vanishes. Moreover, the edge modes form flat bands in the presence of inter-ladder coupling. The original SSH model does not have such a nice property. Second and more importantly, tunnelling in the orbital ladder can form π flux loops and allow time-reversal symmetry breaking, as shown in discussed above. This gives rise to an interesting Z 2 topological insulating state [25] . In contrast, breaking time-reversal symmetry within the SSH model of spinless fermions is impossible because the tunnelling is strictly 1D and thus cannot form flux loops. Finally, we discuss a potential connection of the orbital ladder to Majorana physics [38] , [39] . The orbital ladder at half filling maps to two decoupled Majorana chains (see Supplementary Note 8 ) [22] . Note that the Majorana number is 1 for the double Majorana chains [22] . Topologically protected Majorana fermions with Majorana number −1 (ref. 22 ) can be realized on the orbital ladder using schemes similar to those proposed in [18] , [19] , [20] , [21] , for example, by inducing weak pairing of the form The staggered quantum tunnelling t sp mimics the spin–orbit coupling. For the sp orbital ladder with 2 t s <| μ |<2 t p , we find that the Majorana number is −1 and the resulting Majorana zero modes are topologically protected. The topologically protected Majorana state is a promising candidate for topological quantum computing [40] , [41] . Imaginary transverse tunnelling By rotating individual lattice sites the induced bare coupling term is , where the angular momentum operator is . This term couples the p x to p y orbitals of the B leg. One can tune the rotating frequency to match Ω with the transverse tunnelling t sy from the p y orbital of the B leg to the nearby s orbital on the A leg. Despite the large energy band gap ( ) which separates the p y orbitals from the degenerate s and p x orbitals (bear in mind that the s and p x orbitals are from different legs of the ladder), the low-energy effective Hamiltonian receives a standard second order effect from virtual processes, in which a particle jumps from a p x orbital to the on-site p y orbital and then to the nearby s orbital. The correction is given by , which makes an imaginary transverse tunnelling between nearby s and p x orbitals. Interaction effects To characterize the stability of the topological phase against the inter-orbital interaction H int (see equation (9)), we use the exact diagonalization method to calculate the fidelity metric , where is the ground state wavefunction of the Hamiltonian H = H 0 + H int for a finite chain of length L with N = L fermions. In presence of interaction, the edge states survive as in-gap states (zero energy single particle/hole excitations) [33] . The energy of single particle (hole) excitation is defined as μ p ( μ h ) by μ p = E L +1 − E L ( μ h = E L − E L −1 ), where E N is the ground state energy of the ladder loaded with N fermions. The spatial distribution of the in-gap states is defined as the density profile (Δ n j ) of a hole created out of the ground state, which is where is the ground state with N fermions. The density profile Δ n j is found to be localized on the edges when , and to delocalize when approaching the critical point and finally disappear ( Fig. 2c ). The Mott state appearing at the strong coupling regime has a ferro-orbital order , with ( Fig. 4 ). In our numerical calculation of finite system size, the correlation matrix is calculated and the strength of the ferro-orbital order λ sp is defined as the maximum eigenvalue of [ C ]/ L , extrapolated to the thermodynamic limit. How to cite this article: Li, X. et al . Topological states in a ladder-like optical lattice containing ultracold atoms in higher orbital bands. Nat. Commun. 4:1523 doi: 10.1038/ncomms2523 (2013).